Efficient photoelectrochemical hydrogen production from bismuth vanadate-decorated tungsten trioxide helix nanostructures Tungsten trioxide/bismuth vanadate heterojunction is one of the best pairs for solar water splitting, but its photocurrent densities are insufficient. Here we investigate the advantages of using helical nanostructures in photoelectrochemical solar water splitting. A helical tungsten trioxide array is fabricated on a fluorine-doped tin oxide substrate, followed by subsequent coating with bismuth vanadate/catalyst. A maximum photocurrent density of ~5.35±0.15 mA cm −2 is achieved at 1.23 V versus the reversible hydrogen electrode, and related hydrogen and oxygen evolution is also observed from this heterojunction. Theoretical simulations and analyses are performed to verify the advantages of this helical structure. The combination of effective light scattering, improved charge separation and transportation, and an enlarged contact surface area with electrolytes due to the use of the bismuth vanadate-decorated tungsten trioxide helical nanostructures leads to the highest reported photocurrent density to date at 1.23 V versus the reversible hydrogen electrode, to the best of our knowledge. Photoelectrochemical (PEC) water splitting to produce hydrogen and oxygen has attracted considerable attention since the process was first reported [1] . Various types of semiconductors, such as titanium dioxide (TiO 2 ), haematite (α-Fe 2 O 3 ) and tungsten trioxide (WO 3 ), among others, have been studied for use in this process [2] , [3] . Compared with these single semiconductor electrodes, a heterojunction electrode, which contains two or more dissimilar semiconductors, generally offers more advantages [4] . Among the wide variety of heterojunction systems, tungsten trioxide/bismuth vanadate (WO 3 /BiVO 4 ) has been one of the most studied. The combined properties of WO 3 and BiVO 4 allow this heterojunction system to have a wider range of photon absorption wavelengths due to the relatively narrow band gap of BiVO 4 as well as to provide better charge transfer owing to WO 3 (refs 5 , 6 , 7 ). In general, the structure of a semiconductor electrode has a significant influence on PEC water splitting performance [8] . The current structures used for heterojunction systems are limited to a few configuration types, among which a simple bilayer of the two components is most prevalent [9] . However, some other structures demonstrate advantages over this configuration. For instance, the use of an embedded structure, where one component is encompassed by another, creates a larger contact area for electrons to be transferred more freely, thereby better realizing a synergistic effect in the heterojunction system [10] . To fabricate an embedded structure, the host material should contain free space for the guest material to fill. To date, a variety of nanostructures with large structural voids and surface areas have been fabricated, including nanoparticles, nanorods, nanotubes and nanowires [11] , [12] . One-dimensional linear nanostructures are of tremendous value because they allow electrons/holes to travel from the top to the bottom of the line without changing course, thereby decreasing the travel distance and solving the short electrons/holes diffusion length problem that complicates the use of many semiconductors [13] . Helical structures display this property to some degree by allowing electron/hole transfer along the spiral line; in addition, helices possess a three-dimensional periodic stereostructure with a large surface-to-volume ratio and several unique electrical, mechanical and electromagnetic properties [14] . For these reasons, helical nanostructures have attracted attention and have potential applications in a variety of fields [15] , [16] . In this paper, we present and theoretically characterize BiVO 4 -decorated WO 3 helical nanomaterials for highly efficient PEC water splitting. Few reports exist regarding helical nanostructure use in optical or electrochemical applications, especially concerning their ability to act as a host material in the formation of heterojunction structures for hydrogen production. By optimizing the length of the WO 3 helix (5.5 μm), we achieve a photocurrent density of ~5.35 mA cm −2 at 1.23 V versus the reversible hydrogen electrode (RHE) from the BiVO 4 -decorated WO 3 helix nanostructures. To the best of our knowledge, this value represents the highest photocurrent density reported to date, at 1.23 V versus RHE. Synthesis and characterization The effect of metal doping on the properties of BiVO 4 has been well investigated, with consecutive doping of W and Mo into BiVO 4 ((W, Mo)-BiVO 4 ) resulting in superior photochemical performance [17] , [18] . In this study, (W, Mo)-BiVO 4 was used as a guest material to produce highly efficient PEC cells based on WO 3 helix nanostructures. The principle of operation and experimental details are provided in the experimental section. The crystalline structures of the synthesized helical WO 3 , (W, Mo)-BiVO 4 film and helical WO 3 /(W, Mo)-BiVO 4 heterojunction were confirmed by X-ray diffraction, as shown in Supplementary Fig. 1 . The peaks at 23.3°, 23.8° and 24.6° correspond to the (002), (020) and (200) planes of monoclinic WO 3 , respectively, and the peaks at 28.7° and 30.06° correspond to the (−112) and (040) planes of monoclinic BiVO 4 , respectively [9] . The X-ray photoelectron spectroscopy (XPS) spectra of W and Mo are shown in Supplementary Fig. 2 . Scanning electron microscopy (SEM) images of helical WO 3 and helical WO 3 /(W, Mo)-BiVO 4 are shown in Fig. 1 . 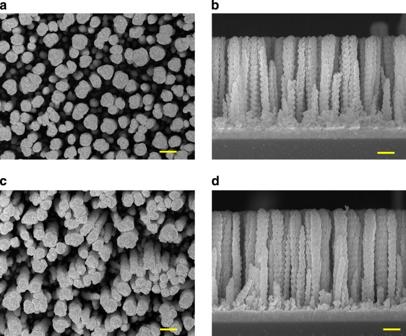Figure 1: Scanning electron microscopy images. (a,b) Top and cross-sectional SEM images of the helical tungsten trioxide (WO3) and (c,d) tungsten trioxide/tungsten, molybdenum-doped bismuth vanadate (WO3/(W, Mo)-BiVO4). From a comparison of the sectional images (b,d), the helical skeleton was well maintained after decoration with (W, Mo)-BiVO4. Scale bar, 1 μm. Figure 1a,b and Fig. 1c,d correspond to helical WO 3 and helical WO 3 /(W, Mo)-BiVO 4 , respectively. As shown in Fig. 1b,d , the helical WO 3 and WO 3 /(W, Mo)-BiVO 4 arrays have similar vertical lengths, suggesting that the (W, Mo)-BiVO 4 film was coated on the lateral surface of the WO 3 helical nanostructure. The surface morphologies of the helical WO 3 and WO 3 /(W, Mo)-BiVO 4 arrays displayed similar characteristics, but the latter had a high packing density, indicating that the (W, Mo)-BiVO 4 covered the WO 3 helices, as shown in Fig. 1a,c . The energy-dispersive X-ray spectroscopy elemental mapping comparisons shown in Supplementary Fig. 3 reveal the uniform distribution of (W, Mo)-BiVO 4 on the helical structure of WO 3 . Figure 1: Scanning electron microscopy images. ( a , b ) Top and cross-sectional SEM images of the helical tungsten trioxide (WO 3 ) and ( c , d ) tungsten trioxide/tungsten, molybdenum-doped bismuth vanadate (WO 3 /(W, Mo)-BiVO 4 ). From a comparison of the sectional images ( b , d ), the helical skeleton was well maintained after decoration with (W, Mo)-BiVO 4 . Scale bar, 1 μm. 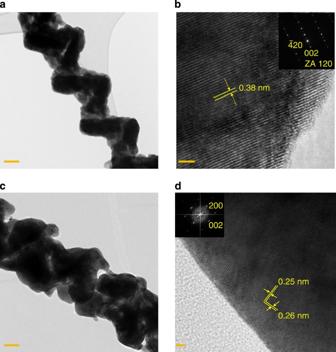Figure 2: Transmission electron microscopy images. TEM images of the helical WO3(a) showing the three-dimensional helical nanostructure and (c) the decoration with (W, Mo)-BiVO4. HR-TEM images and corresponding selected area electron diffraction patterns of (b) a helical WO3and (d) WO3/(W, Mo)-BiVO4. Fromc, it can be confirmed that (W, Mo)-BiVO4uniformly covered the entire surface of the helical WO3, and the ordered helical arrangement was maintained. Fromb, ad-spacing of 0.38 nm was obtained, which could be assigned to the (002) plane of WO3; fromd,d-spacings of 0.25 and 0.26 nm were obtained, which correspond to the (002) and (200) planes, respectively, of monoclinic BiVO4. Scale bar, 100 nm (a,c) and 2 nm (b,d). Full size image Figure 2a,c show transmission electron microscopy (TEM) images of helical WO 3 and WO 3 /(W, Mo)-BiVO 4 , respectively, and corresponding high-resolution TEM (HR-TEM) images with diffraction patterns are shown in Fig. 2b,d . The spot diffraction patterns and the pronounced diffraction contrast of the HR-TEM image in Fig. 2b indicate the high crystallinity of the helical WO 3 . It is observed in Fig. 2c that (W, Mo)-BiVO 4 uniformly covers the entire surface of the helical WO 3 , as further confirmed by linear elemental detection ( Supplementary Fig. 4 ). HR-TEM images and corresponding selected area electron diffraction patterns showed d -spacings of 0.38 nm, which can be assigned to the (002) plane of helical WO 3 ( Fig. 2b ), and of 0.25 and 0.26 nm, corresponding to the (002) and (200) planes of monoclinic BiVO 4 ( Fig. 2d ), respectively. Dark-field TEM images with separate diffraction spots for the helical WO 3 ( Supplementary Fig. 5 ) indicated that the WO 3 helixes were composed of a large near-single crystalline domain with a few grain boundaries. The large grain size coupled with the near-single crystallinity of the WO 3 helixes ensures that carrier transport through the WO 3 helixes will be enhanced significantly in comparison with that through a network of nanoparticles, where the grain boundaries between the nanoparticles act as recombination and scattering centres for carrier transport. Figure 2: Transmission electron microscopy images. TEM images of the helical WO 3 ( a ) showing the three-dimensional helical nanostructure and ( c ) the decoration with (W, Mo)-BiVO 4 . HR-TEM images and corresponding selected area electron diffraction patterns of ( b ) a helical WO 3 and ( d ) WO 3 /(W, Mo)-BiVO 4 . From c , it can be confirmed that (W, Mo)-BiVO 4 uniformly covered the entire surface of the helical WO 3 , and the ordered helical arrangement was maintained. From b , a d -spacing of 0.38 nm was obtained, which could be assigned to the (002) plane of WO 3 ; from d , d -spacings of 0.25 and 0.26 nm were obtained, which correspond to the (002) and (200) planes, respectively, of monoclinic BiVO 4 . Scale bar, 100 nm ( a , c ) and 2 nm ( b , d ). Full size image The ultraviolet–visible absorbance spectra of the helical WO 3 and WO 3 /(W, Mo)-BiVO 4 are shown in Supplementary Fig. 6 . In the absorption spectrum of the helical WO 3 sample, one sharp near-bandgap absorption edge at 2.8 eV (~440 nm), corresponding to the band gap value of WO 3 , can be observed. By contrast, the absorption edge of WO 3 /(W, Mo)-BiVO 4 at ~510 nm, which is red-shifted from the 2.8 eV absorption edge, can probably be attributed to the absorption caused by (W, Mo)-BiVO 4 . PEC performances PEC measurements, including current density–voltage ( J–V ) curves, incident-photon-to-current efficiency (IPCE) and gas evolution measurements, were carried out under AM1.5G light. In this study, we were able to control the length of the helical WO 3 from 1 to 7.5 μm. As shown in Supplementary Fig. 7 , the best PEC performances of pure WO 3 helix were observed at a length of 5.5 μm. Thus, all the WO 3 /(W, Mo)-BiVO 4 samples were based on 5.5-μm-length WO 3 helix arrays. As shown in Fig. 3a , the current density over the helical WO 3 /(W, Mo)-BiVO 4 heterojunction exceeded 3.9 mA cm −2 at 1.23 V versus RHE when measured in 0.5 M Na 2 SO 4 adjusted to pH 7 with buffer solution. Here we also estimated the charge separation efficiency for our heterojunction system by evaluating its sulphite oxidation performance ( J SUL ). It is known that for each single or heterojunction semiconductor, the maximum photocurrent density ( J MAX ) is determined by its band gap energy, but the PEC performances are influenced by its light harvesting efficiency ( η LHE ), charge separation efficiency ( η SEP ) and the surface transfer efficiency ( η TRA ) [19] , [20] . For sulphite oxidation, η TRA can be considered to be 100% due to its fast oxidation kinetics, resulting in J SUL = J MAX × η LHE × η SEP (ref. 21 ). The value of η SEP can be obtained by dividing J SUL by ( J MAX × η LHE ). The detailed calculation of J MAX and η LHE for our helical WO 3 /(W, Mo)-BiVO 4 heterojunction is illustrated in the Supplementary Fig. 8 and the final integration result of J MAX × η LHE gave a value of 6.27 mA cm −2 . Moreover, the curve of J SUL for the helical WO 3 /(W, Mo)-BiVO 4 is shown in Supplementary Fig. 9a . By dividing Supplementary Fig. 9a by 6.27, over 94% separation efficiency was obtained at 1.23 V versus RHE ( Supplementary Fig. 9b ). This result demonstrates that the metal doping of BiVO 4 as well as the use of a compact interface between WO 3 and BiVO 4 enabled by the unique helical nanostructure of the host material led to a significantly enhanced charge separation efficiency for the photoanode. 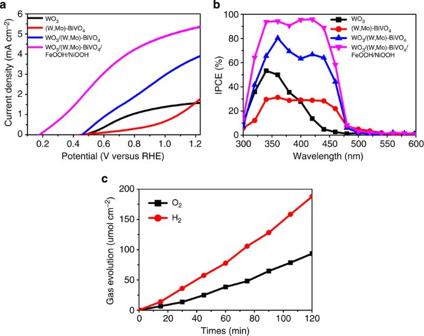Figure 3: Photoelectrochemical performances. J–V(a) and IPCE (b) curves of helical WO3, (W, Mo)-BiVO4, WO3/(W, Mo)-BiVO4and WO3/ (W, Mo)-BiVO4/ FeOOH/NiOOH measured in 0.5 M K2SO4in phosphate buffer (pH 7) under AM 1.5 G, 100 mW cm−2illumination; the pure (W, Mo)-BiVO4has a considerably lower current density compared with WO3under 1.23 V versus RHE. (c) Gas evolution behaviour over time. Optimized helical WO3/(W, Mo)-BiVO4/FeOOH/NiOOH was used in a two electrode configuration under 1.2 V. During the gas evolution process, the average photocurrent density was ~2.6 × 10−3A, which can be used for the estimation of the faradaic efficiency for oxygen/hydrogen evolution (seeSupplementary Methods). Figure 3: Photoelectrochemical performances. J–V ( a ) and IPCE ( b ) curves of helical WO 3 , (W, Mo)-BiVO 4 , WO 3 /(W, Mo)-BiVO 4 and WO 3 / (W, Mo)-BiVO 4 / FeOOH/NiOOH measured in 0.5 M K 2 SO 4 in phosphate buffer (pH 7) under AM 1.5 G, 100 mW cm −2 illumination; the pure (W, Mo)-BiVO 4 has a considerably lower current density compared with WO 3 under 1.23 V versus RHE. ( c ) Gas evolution behaviour over time. Optimized helical WO 3 /(W, Mo)-BiVO 4 /FeOOH/NiOOH was used in a two electrode configuration under 1.2 V. During the gas evolution process, the average photocurrent density was ~2.6 × 10 −3 A, which can be used for the estimation of the faradaic efficiency for oxygen/hydrogen evolution (see Supplementary Methods ). Full size image By comparing the photocurrent values of the helical WO 3 /(W, Mo)-BiVO 4 for water oxidation and sulphite oxidation, as shown in Fig. 3 and Supplementary Fig. 9a , it was observed that the surface recombination of the WO 3 /(W, Mo)-BiVO 4 photoanode was still an obstacle for water oxidation. To obtain the best performance from the helical WO 3 /(W, Mo)-BiVO 4 photoanode system, we also evaluated the incorporation of surface oxygen evolution catalyst (OEC) layers in the WO 3 /(W, Mo)-BiVO 4 photoanode to improve its water oxidation kinetics. It is well known that cobalt-phosphate (Co-Pi) [22] , Pt [23] and the newly reported FeOOH/NiOOH [24] are the most widely applied OEC layers. Here we evaluated each of these materials to obtain the best performance from our heterojunction system. All three surface catalysts were optimized by controlling the deposition time on the surface of the WO 3 /(W, Mo)-BiVO 4 photoanode (the optimal deposition time for each catalyst is described in the experimental section). The relative XPS spectra of Co, P, Pt, Fe and Ni are shown in Supplementary Fig. 2 and comparisons of the corresponding PEC performances are shown in Supplementary Fig. 10 . Moreover, the dark current behaviours of all the photoanodes are provided in Supplementary Fig. 11 . It can be observed that under the optimized conditions, the catalyst FeOOH/NiOOH showed a more negative flat band potential after modification as well as the highest oxygen evolution reaction activities with a strong negative shift in the onset potential, indicating that it can suppress surface recombination [24] . This resulted in a higher photocurrent density at both low and high potentials, as well as the highest current density of 5.35±0.15 mA cm −2 at 1.23 V versus RHE for water oxidation, as shown in Fig. 3a (the independent runs and error bars for the highest current density are shown in Supplementary Fig. 12 ). The monochromatic IPCE data at 1.23 V versus RHE for the helical WO 3 , the (W, Mo)-BiVO 4 thin film, the helical WO 3 /(W, Mo)-BiVO 4 and the helical WO 3 /(W, Mo)-BiVO 4 /FeOOH/NiOOH at their best performance are shown in Fig. 3b , and the helical WO 3 /(W, Mo)-BiVO 4 /FeOOH/NiOOH demonstrated tremendously high IPCE values of over 90%. Note that in the IPCE data there is no noticeable variation in ultraviolet–visible absorption behaviour between WO 3 /(W, Mo)-BiVO 4 and WO 3 /(W, Mo)-BiVO 4 /FeOOH/NiOOH, which demonstrates that the FeOOH/NiOOH modification did not interfere with the light absorption of WO 3 /(W, Mo)-BiVO 4 ( Supplementary Fig. 6 ). The characterization of gas evolution is critical to developing successful applications of WO 3 /BiVO 4 heterojunctions, but it has rarely been explored in previous reports. Herein, the hydrogen and oxygen evolution from helical WO 3 /(W, Mo)-BiVO 4 /FeOOH/NiOOH under optimal conditions at an external potential of 1.2 V was characterized using a two-electrode configuration, as shown in Supplementary Fig. 13 . The gas evolution as a function of the irradiation time is shown in Fig. 3c . From these data, an overall faradaic efficiency of ~96.21% for oxygen evolution was estimated; the detailed calculation process is shown in the Supplementary Methods . The very weak faradaic loss can be ascribed to side reactions occurring at the photoanode and to the inhibition of proton reduction, as well as possible recombination events at the counter electrode [25] , [26] . Meanwhile, the long-term stability of the WO 3 /(W, Mo)-BiVO 4 /FeOOH/NiOOH heterojunction sample was checked to confirm the possibility for its commercialization ( Supplementary Fig. 14 ), and the decline of the performance was qualified with detailed discussions. In this study, we have compared the variation by looking at the difference between the hourly observed photocurrent densities for each day. We assumed that the PEC was operated during the daytime (12 h) for each day. In summary, for the PEC field, although WO 3 /BiVO 4 heterojunction systems are relatively conventional, our study improved this system by employing a helical host material (WO 3 ) decorated with a guest material (BiVO 4 ). The structural novelty and superior properties of this material are reflected in its high photocurrent density, as well as in the high photon-to-current conversion efficiency and in the significant hydrogen and oxygen generation, and we can conclude that the helical structure used as the framework of the system plays a crucial role in improving the system performance. In addition to the improvements in charge separation and transportation enabled by the microstructural characteristics of the helical WO 3 , as observed by TEM measurements, the unique three-dimensional helix array can change the optical properties of WO 3 dramatically, particularly its light scattering and absorption. To investigate the effect of the helical nanostructure on light scattering, finite elemental simulations were performed using commercial software COMSOL multiphysics with the wave optics module. Theoretical background, structural and optical details of the simulations are provided in Supplementary Table 1 . 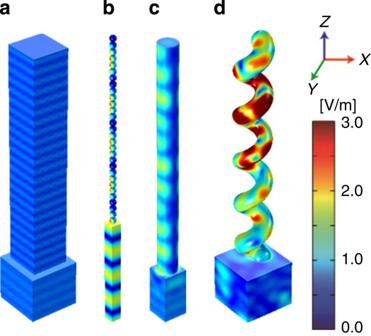Figure 4: Schemes of the electric field magnitude for various nanostructures. Distribution of the electric field magnitude at the WO3surface of (a) a thin film (2.4 μm height), (b) a stack of nanoparticles (30 nm diameter, 30 nanoparticles), (c) a nanorod (100 nm rod diameter, 2.4 μm height) and (d) a nanohelix (100 nm rod diameter, 400 nm helix diameter, 2.4 μm height). Anx-polarized electric field of a plane wave with a 450-nm wavelength was normally incident from the top. The periodic boundary conditions were 50 nm × 50 nm for the stack of nanoparticles, 250 nm × 250 nm for the nanorod and 550 nm × 550 nm for the thin film and the nanohelix structures. All structures were on a 500-nm F:SnO2(FTO) film. The refractive indices of air, WO3, F:SnO2and glass used for this simulation were 1.00, 2.10, 1.74 and 1.50, respectively. The scale bar on the right represents the magnitude of the electric field. Figure 4 shows the distribution of the magnitude of the electric field, as indicated by the colour scale, at the surfaces of various WO 3 nanostructures ( a . a thin film, b . a stack of nanoparticles, c . a nanorod [21] , d . a nanohelix) when an x -polarized electric field of a plane wave with a 450-nm wavelength is normally incident from the top. The magnitudes of the electric fields inside the WO 3 thin film, the stack of nanoparticles and the nanorod show wave-guide-like periodic profiles caused by interference between the incident and reflected waves with negligible scattering effects. The relatively higher magnitude of the electric field for the stack of nanoparticles than for the thin film and the nanorod is due to the reduced effective refractive index caused by the combination of the WO 3 nanoparticles and the air medium, which results in negligible scattering because the nanoparticles are much smaller than the wavelength of light [27] . However, a much more complex distribution of the electric field with an ~3-fold higher amplitude than that of the other structures is observed for the three-dimensional nanohelices due to their greater light-scattering cross-section. Video clips showing time-dependent propagation of electric fields through the various WO 3 nanostructures are presented in Supplementary Movies 1–4 . Figure 4: Schemes of the electric field magnitude for various nanostructures. Distribution of the electric field magnitude at the WO 3 surface of ( a ) a thin film (2.4 μm height), ( b ) a stack of nanoparticles (30 nm diameter, 30 nanoparticles), ( c ) a nanorod (100 nm rod diameter, 2.4 μm height) and ( d ) a nanohelix (100 nm rod diameter, 400 nm helix diameter, 2.4 μm height). An x -polarized electric field of a plane wave with a 450-nm wavelength was normally incident from the top. The periodic boundary conditions were 50 nm × 50 nm for the stack of nanoparticles, 250 nm × 250 nm for the nanorod and 550 nm × 550 nm for the thin film and the nanohelix structures. All structures were on a 500-nm F:SnO 2 (FTO) film. The refractive indices of air, WO 3 , F:SnO 2 and glass used for this simulation were 1.00, 2.10, 1.74 and 1.50, respectively. The scale bar on the right represents the magnitude of the electric field. Full size image To experimentally verify the enhanced light scattering from the three-dimensional WO 3 nanohelix array, both the specular and diffuse reflectance from an ~6-μm WO 3 thin film and from the nanohelix array were measured, as shown in Fig. 5b . A monochromatic 450-nm light beam was incident to the top part of the thin film and the nanohelix array with a 30° angle of incidence (AOI) and the reflected light was measured by scanning a photodetector with an angle of detection (AOD), as schematically shown in Fig. 5a . Although the specular reflectance (when AOD≈AOI) of the thin film structure was significantly higher than the diffuse reflectance (when |AOD-AOI|≥7°), diffuse reflectance was dominant with almost no specular reflectance peak for the WO 3 nanohelices, as shown in Fig. 5b . This indicates that the nanohelix structure can capture much larger amount of light due to strong light scattering than the thin film can, which is consistent with our simulation results. Based on our microstructural and optical characterizations of the helical WO 3 array, we believe that the enhanced PEC performance of the BiVO 4 -decorated WO 3 helix nanostructures can be attributed to two important sequential improvements: first, a boost in the number of photo-generated carriers due to strong light scattering, and second, the very efficient separation and transportation of photo-generated carriers at the large BiVO 4 -WO 3 interface and through the near-single crystalline WO 3 nanohelix structures, respectively. 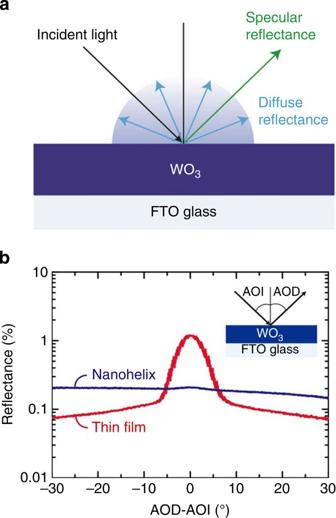Figure 5: Light-scattering effect and the relative reflectance spectrum. (a) A schematic of specular and diffuse reflectance and (b) the specular and diffuse reflectance of a 6-μm WO3thin film and of the nanohelix array as a function of the difference between the angle of the detector and the angle of incidence (30°). The inset shows the schematic measurement configuration. Figure 5: Light-scattering effect and the relative reflectance spectrum. ( a ) A schematic of specular and diffuse reflectance and ( b ) the specular and diffuse reflectance of a 6-μm WO 3 thin film and of the nanohelix array as a function of the difference between the angle of the detector and the angle of incidence (30°). The inset shows the schematic measurement configuration. Full size image The advantages of the helical structures mentioned above were used to produce significantly enhanced photoanode performance. In the current study, by using the heterojunction of two semiconductors in a helical structure, we obtained a photocurrent that surpasses this value. Furthermore, this value represents the highest current density reported for two semiconductors in an n–n heterojunction system in a neutral solution. The results show that this nanohelix is an excellent option for PEC applications and is comparable to other nanostructures. In this work, we fabricated, characterized and analysed a helical heterojunction structure. In particular, this material’s promising application in PEC water splitting was investigated. We also employed a heterojunction system with proper doping and surface modification methods to optimize the system’s performance as a photoanode. The highest photocurrent density of this system reached ~5.35 mA cm −2 at 1.23 V versus RHE, and significant gas evolution was triggered using this system compared with other planar thin film photoanodes. These results demonstrate that our helical structure possesses many excellent properties, including strong light-scattering effects for enhanced light harvesting and an appropriate radius, and large surface area for charge separation as well as near single crystallinity for effective charge transport, which are advantageous in PEC water splitting. In addition, diffusion of W from WO 3 into BiVO 4 forming a gradient doping of W, known to be beneficial for the charge separation [28] , can be facilitated by large interface area between WO 3 nanohelixes and BiVO 4 . We observed the diffusion of W atoms and formation of a gradient of W atoms in BiVO 4 using synchrotron radiation photoemission spectroscopy, and summarized the results in the Supplementary Fig. 15 . A main requirement in PEC cells that can induce spontaneous H 2 and O 2 evolution simultaneously with a single semiconductor photoelectrode is the discovery of a material that have appropriate bandgap about 2.5 eV, with a conduction band sufficiently negative for H 2 evolution and the valence band sufficiently positive for O 2 evolution. Unfortunately, the device with spontaneous gas evolution could not have high efficiency because the semiconductor with 2.5 eV need additional bias for efficient charge separation. As far as we know, one of best approaches for solving this problem of single or heterojunction semiconductor based PEC cells is using tandem device configuration. In fact, our samples with the 5.5-μm thickness have weak transparency; hence, we did not consider using it in a photoanode/photovoltaic tandem cell. However, there is the previous report mentioned the photovoltaic/photoanode tandem cell in which the photovoltaic (such as a dye-sensitized solar cell (DSSC)) is placed in front of the photoanode [29] . Although the performance is not best compared with other kinds of configurations, it still shows potential application in the future. In this configuration, the low transmittance and the high light-scattering effect of the photoanode will not be a problem for the overall performance of the tandem cell. In addition, we also have to consider the preparation of more transparent photoanode with helix nanostructures for conventional photoanode/photovoltaic tandem cells. In this study, we only tried to show the best performances of conventional photoanode itself for PEC application. Finally, as the model simulation does not rely on the WO 3 /BiVO 4 system and is not confined to PEC water splitting, it is reasonable to hypothesize that our research can be applied to the use and analysis of novel nanostructures made from various materials in photovoltaic, solar or other photo-to-electrical cells. Fabrication of helically nanostructured WO 3 Oblique angle deposition has been widely used in the fabrication of ordered nanostructure arrays and offers numerous advantages, such as control over thickness/shape, reproducibility and low cost [30] , [31] . In this study, the F:SnO 2 (FTO) substrate size was 1.5 cm × 1.5 cm. The active region (1.5 cm × 1 cm) was defined with a shadow mask. Tungsten oxide powder (WO 3 , Taewon Scientific Co.) was placed in a carbon crucible and subjected to e-beam evaporation. Before helix fabrication, a thin WO 3 film (~50 nm) was first deposited by e-beam coating. Then, the substrate was spun for 2 s at 1 r.p.m. and then stopped for 12 s with an 80° oblique angle and a 3.5 Å s −1 deposition rate to fabricate the helix arrays. The pressure in the chamber was maintained at 1.5 × 10 −6 Torr. The as-deposited samples were annealed at 500 °C for 1 h. Preparation of the (W, Mo)-BiVO 4 precursor solution The preparation of the (W, Mo)-BiVO 4 precursor solution was accomplished using the following method [17] . Bismuth nitrate pentahydrate (BiN 3 O 9 · 5H 2 O, 99.99%, Aldrich), ammonium paratungstate ((NH 4 ) 10 H 2 (W 2 O 7 ) 6 )), 99.99%, Aldrich), Vanadium(III) chloride, (VCl 3 , 99%, Alfa-Aeser) and ammonium molybdate tetrahydrate ((NH 4 ) 6 Mo 7 O 24 · 4H 2 O, 99.98%, Aldrich) were used as the Bi, W, V and Mo sources, respectively. Solutions of 2.2 mM Bi(NO 3 ) 3 · 5H 2 O, 2.5 mM VCl 3 , 8 μM (NH 4 )10H 2 (W 2 O 7 ) 6 · x H 2 O and 43 μM (NH 4 ) 6 Mo 7 O 24 · 4H 2 O dissolved in ethylene glycol were prepared. Fabrication of the (W, Mo)-BiVO 4 and WO 3 /(W, Mo)-BiVO 4 The WO 3 /(W, Mo)-BiVO 4 heterojunction electrode was fabricated by slowly dropping 150 μl aliquot of the precursor solution onto the surface of the helical WO 3 , which was the optimal volume for a 1.5 cm × 1.5 cm-sized FTO with 5.5 μm WO 3 helices. For making pure (W, Mo)-BiVO 4 electrode, same amount of precursor was used to drop onto the top of cleaned FTO glass with 1.5 cm × 1.5 cm size. Next, the samples were annealed at 500 °C for 3 h following a temperature increase from room temperature to 500 °C over the course of 8 h, resulting in sufficient crystallization and full densification. Surface modification by the OEC layer In case of Co-Pi, the precursor was prepared from cobalt (II) nitrate hexahydrate (CoN 2 O 6 · 6H 2 O, 99.9%, Aldrich) and potassium phosphate buffer (0.5 M, Sigma-Aldrich) using a Co/P molar ratio of 1:200. After the fabrication of the WO 3 /(W, Mo)-BiVO 4 heterojunction, the sample was placed into the Co-Pi precursor solution for photo-assisted electrodeposition. The potential was +1.1 V versus Ag/AgCl illuminated under 1 sun and AM 1.5 G conditions [20] . The optimum deposition time was 5 min. In case of Pt, a 10-mM H 2 PtCl 6 · 6H 2 O (Chloroplatinic Acid, Aldrich) solution in deionized water was first prepared and the sample was immersed into the solution for photodeposition with illumination under 1 sun and AM 1.5 G conditions. The optimum deposition time was 15 min. In case of FeOOH/NiOOH, an FeOOH layer was first photodeposited (1 sun, AM 1.5 G) using a 0.1-M FeSO 4 (iron(II) sulphate heptahydrate, 99%, Aldrich) solution, during which an external bias of 0.25 V versus Ag/AgCl was applied. Next, the sample was placed into 0.1 M NiSO 4 (nickel(II) sulphate hexahydrate, 99%, Aldrich, adjusted pH to 6.7 with basic solution) for photodeposition (1 sun, AM 1.5 G) with an external bias of 0.11 V versus Ag/AgCl. Finally, NiOOH was electrodeposited in 0.1 M NiSO 4 by applying 1.2 V versus Ag/AgCl to fully cover the surface of the electrode. The optimum deposition time was 13 min for FeOOH photodeposition, 6 min for NiOOH photodeposition and 90 s for the final electrodeposition. All of the catalyst precursor solutions were purged with nitrogen gas for at least 45 min before use. Analyses The PEC performances were measured using a potentiostat (CH Instrument, CHI 660) in a three-electrode optical cell, in which the reference electrode was Ag/AgCl and the counter electrode was Pt foil. For water oxidation, the electrolyte was a 0.5 M K 2 SO 4 (Potassium sulphate, 99%, Aldrich) solution adjusted to pH 7 with potassium phosphate buffer. For sulphite oxidation, the electrolyte was 1 M K 2 SO 3 (Potassium sulphite, 90%, Aldrich) in phosphate buffer and the final pH was ~7.5. A solar simulator (Peccell, Yokohama, Japan, PEC-L01) was used as the light source, which provided 1 sun and AM 1.5 G simulated sunlight. To calibrate the light intensity, a silicon reference cell (Fraunhofer ISE, Certificate No.C-ISE269) was used. The IPCE was confirmed using a monochromator (Polaronix K3100 IPCE Measurement System, McScience) with a 300-W xenon light source. For the gas evolution process a quartz reactor is used, which is sealed by the rubber plugs and parafilms. The sample and Pt are placed in the reactor in the two-electrode configuration with 1.2 V absolute bias. The positions for leads to get through the rubber plug are also sealed by super glue and parafilm. Before reaction and total sealing process, the electrolyte (0.5 M K 2 SO 4 , adjust to pH 7 with phosphate buffer) and the whole space in the reactor are purged via nitrogen gas. The silicon reference cell (Fraunhofer ISE, Certificate No.C-ISE269) was used to calibrate the light intensity. During reaction, the gas will be extracted by the glass injection syringe every 15 min for the analysis by gas chromatograph (Agilent Technologies 7890A GC system, made in USA) with a 5-Å molecular sieve column [24] , [32] . X-ray diffraction measurements were conducted using a Siemens diffractometer D500/5000 in the Bragg–Bretano geometry. XPS data were obtained using an AESXPS instrument (ESCA2000 from VG Microtech in England). SEM and energy-dispersive X-ray mapping, as well as TEM and HR-TEM, were performed using a field-emission SEM (JSM-7000F, Japan) and a JEOL JEM-2100F (Japan) electron microscope, respectively. Synchrotron radiation photoemission spectroscopy measurements were performed to investigate the diffusion of W in WO 3 helixes into BiVO 4 layer using 4D beamline of Pohang Accelerator Laboratory, South Korea. Pure BiVO 4 (without W and Mo doping) coated on WO 3 nanohelix array were prepared and depth profiling of chemical components was performed by carrying out repeated processes of synchrotron radiation photoemission spectroscopy measurements and Ar ion sputtering. Photon energy of 200 eV was chosen due to much larger photoionization cross-section of W-4f than other elements. How to cite this article : Shi, X. et al . Efficient photoelectrochemical hydrogen production from bismuth vanadate-decorated tungsten trioxide helix nanostructures. Nat. Commun. 5:4775 doi: 10.1038/ncomms5775 (2014).